A red-shifted fluorescent substrate for aldehyde dehydrogenase Selection of cells positive for aldehyde dehydrogenase (ALDH) activity from a green-fluorescent background is difficult with existing reagents. Here we report a red-shifted fluorescent substrate for ALDH, AldeRed 588-A , for labelling viable ALDH pos cells. We demonstrate that AldeRed 588-A successfully isolates ALDH hi human haematopoietic stem cells from heterogeneous cord blood mononuclear cells. AldeRed 588-A can be used for multicolour applications to fractionate ALDH pos cells in the presence of green fluorophores including the ALDEFLUOR reagent and cells expressing enhanced green-fluorescent protein (eGFP). AldeRed 588-A stains ALDH pos murine pancreatic centroacinar and terminal duct cells, as visualized using fluorescent microscopy. AldeRed588-A provides a useful tool to select stem cells or study ALDH within a green-fluorescent background. Aldehyde dehydrogenase (ALDH) is an evolutionarily conserved enzyme with pyridine nucleotide-dependent oxidoreductase activity that performs a variety of critical cellular processes [1] . These include production of retinoic acid essential for mammalian development [2] , metabolism of fats and amino acids and detoxification of endogenous and exogenous sources of hazardous aldehyde byproducts [3] . Twenty human ALDH genes have been identified and many of their functions are still unknown [4] . For the past two decades ALDH has been studied as a potential universal marker for normal and cancer stem cells, as certain isoenzymes of the ALDH superfamily have been identified as key elements of these cells [5] . For example, Aldh1a1 and Aldh3a1 have been implicated in the protection of stem cells from cytotoxic drugs. ALDH pos stem cells have been used as resources for regenerative medicine in preclinical models [6] and in an ongoing clinical trial for ischaemic cardiomyopathy (clinicaltrial.gov, NCT00314366). ALDH1 has been identified as a marker used to isolate cancer stem cells of various human malignancies including bladder, breast, cervical, colon, head and neck, liver, lung, pancreas, prostate and ovary [5] . Recently Gerber et al. [7] showed that the presence of leukemic stem cells with intermediate ALDH activity (ALDH int ) could be used as a predictor for relapse after therapy, whereas normal haematopoietic stem cells (HSCs) retain high ALDH activity. Since these normal and cancer stem cells are very rare, methods to identify and isolate viable, functionally active ALDH pos cells are needed to characterize or utilize them. The ALDEFLUOR reagent (Aldagen Inc., Durham, NC, USA) has enabled the primary commercial assay used today for isolation of viable ALDH pos cells, which was patterned after the original dansyl aminoacetaldehyde-based assay developed by Jones et al. [8] Although very sensitive and specific for staining viable ALDH pos cells, as it emits in the green region of the electromagnetic spectrum (512 nm), the ALDEFLUOR reagent cannot be simultaneously utilized in cells or mice expressing green-fluorescent proteins [9] , [10] . This has limited the use of many valuable cell and animal models with green-fluorescent signals to study ALDH, and there have been increasing demands for non-green functional ALDH markers. Here we report the synthesis, in vitro validation and applications of a red-shifted fluorescent substrate of ALDH. Syntheses of candidate ALDH substrates We synthesized three candidate substrates of ALDH containing fluorophores that emit in the red region of the spectrum ( Fig. 1 ). Three red fluorophores, ( E )-4-(4-(dimethylamino)styryl)-1-(3-isothiocyanatopropyl)pyridin-1-ium chloride 1 , BODIPY 576/589 succinimidyl ester 2 and BODIPY 650/665 succinimidyl ester 3 were conjugated to aminoacetaldehyde diethyl acetal to produce diethyl acetals 4 , 5 , 6 , which were purified using reverse phase liquid chromatography or flash column chromatography. Maximum excitation and emission wavelengths for 4 , 5 and 6 were 493/590, 588/599 and 659/671 nm, respectively ( Supplementary Fig. 1 ). Acid hydrolysis of the diacetals to produce the corresponding aldehydes, AldeRed 493-A , AldeRed 588-A and AldeRed 659-A , was performed immediately before the assay. 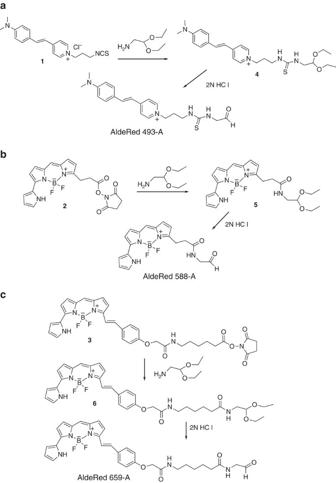Figure 1: Synthesis of candidate red-shifted fluorescent substrates for ALDH. (a)AldeRed 493-A, (b)AldeRed 588-A, (c)AldeRed 659-A. Each compound was prepared as the diacetal (4,5and6) and deprotected to the aldehyde before use. Figure 1: Synthesis of candidate red-shifted fluorescent substrates for ALDH. ( a ) AldeRed 493-A , ( b ) AldeRed 588-A , ( c ) AldeRed 659-A . Each compound was prepared as the diacetal ( 4 , 5 and 6 ) and deprotected to the aldehyde before use. Full size image In vitro validation of candidate ALDH substrates We tested the ALDH specificity of the three candidate substrates using human and murine cell lines that express different levels of ALDH, namely K562 (ALDH hi ), L1210 (ALDH low ) and L1210/cpa (ALDH hi ) [11] . We analysed cell uptake and retention of the substrates in the absence and presence of the ALDH inhibitor, diethylaminobenzaldehyde (DEAB) [8] . As with the original ALDEFLUOR reagent, it is the acid-deprotected aldehyde form of the candidate substrate that diffuses into cells and is converted into the corresponding carboxylate by ALDH, which is retained. Substrates were evaluated using the LSR II (BD Biosciences, San Jose, CA, USA) fluorescence-activated cell sorter (FACS) equipped with four lasers and 14 emission filters (Methods and Supplementary Figs 2–4 ). Of the three compounds tested, AldeRed 588-A demonstrated specific uptake for both K562 and L1210/cpa cells when compared with the DEAB-treated control, indicating ALDH substrate specificity ( Fig. 2a ). All three substrate candidates stained cells as indicated by shifted signals in selected emission filter sets compared with unstained cells ( Supplementary Figs 2–4 ). However, AldeRed 493-A did not demonstrate increased signals for either ALDH pos cell line, and AldeRed 659-A exhibited only a minimal shift of fluorescent uptake in comparison with DEAB-treated control ( Fig. 2a and Supplementary Figs 2–4 ). We were able to use the basic analytical FACS device, FACSCalibur (BD Biosciences), with its single blue laser, to detect the cellular uptake of AldeRed 588-A using the FL2 filter ( Supplementary Fig. 5 ). To examine further AldeRed 588-A as a substrate for ALDH, we compared the ability of the ALDEFLUOR reagent and AldeRed 588-A for detecting different levels of ALDH expression. We stained L1210 (ALDH low ) and L1210/cpa (ALDH hi ) cells and found that both reagents were able to differentiate these two cell lines ( Fig. 2b ). As further confirmation, we performed co-staining with the ALDEFLUOR reagent and AldeRed 588-A . Both substrates proportionately co-stained ALDH hi K562 and L1210/cpa cell lines ( Fig. 2c ). Importantly, these data demonstrate that red-fluorescent AldeRed 588-A could be used for co-staining with green fluorophores. 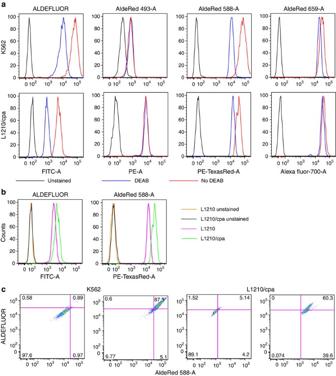Figure 2: AldeRed 588-A is a specific substrate for ALDH. (a) Fluorescent candidates and the ALDEFLUOR reagent were tested with K562 and L1210/cpa cells. Thexaxis represents selected detection filters of the LSR II FACS system. (b)AldeRed 588-Aand the ALDEFLUOR reagent tested with L1210/cpa and L1210 cells. (c) Co-staining of K562 and L1210/cpa cells withAldeRed 588-Aand the ALDEFLUOR reagent. DEAB: diethylaminobenzaldehyde. Figure 2: AldeRed 588-A is a specific substrate for ALDH. ( a ) Fluorescent candidates and the ALDEFLUOR reagent were tested with K562 and L1210/cpa cells. The x axis represents selected detection filters of the LSR II FACS system. ( b ) AldeRed 588-A and the ALDEFLUOR reagent tested with L1210/cpa and L1210 cells. ( c ) Co-staining of K562 and L1210/cpa cells with AldeRed 588-A and the ALDEFLUOR reagent. DEAB: diethylaminobenzaldehyde. Full size image Isolation of ALDH hi human HSCs Primitive adult stem cells are rare, suggesting that a single-step isolation method would be useful to maximize the efficiency of purification and minimize damage to cells. We tested AldeRed 588-A for its capacity to isolate ALDH hi stem cells from a heterogeneous mixture of cells in human cord blood. We labelled mononuclear cells derived from human cord blood with ALDEFLUOR and isolated the ALDH hi cell population that is not present in cells treated with DEAB (control; Fig. 3a ). Isolated cells were capable of giving rise to multiple types of differentiated colonies including BFU-E (burst forming unit-erythroid), CFU-G (colony forming unit-granulocyte), CFU-M (colony forming unit-megakaryocyte), CFU-GM (colony forming unit-granulocyte, monocyte) and CFU-GEMM (colony forming unit-granulocyte, erythrocyte, monocyte, megakaryocyte; Table 1 and Supplementary Fig. 6 ) indicating that these ALDH hi cells are enriched HSCs. We asked whether AldeRed 588-A could perform the same task as ALDEFLUOR. AldeRed 588-A successfully isolated ALDH hi populations ( Fig. 3b ), which gave rise to differentiated colonies in a very similar pattern to cells isolated by ALDEFLUOR ( Table 1 and Supplementary Fig. 6 ). We then co-labelled human cord blood mononuclear cells with ALDEFLUOR and AldeRed 588-A to determine whether both agents were staining the same HSC populations. We confirmed that cells labelled green and red represented identical ALDH hi populations that could be isolated by gating them into their respective channels by FACS ( Fig. 3c,d ). In addition, cells exhibited proportional staining patterns for both reagents indicating specificity of the staining ( Supplementary Fig. 7 ). These results indicate that AldeRed 588-A can efficiently stain and isolate ALDH hi HSCs among heterogeneous cell populations and can be used with green ALDEFLUOR to increase the purity of ALDH pos cells, if necessary. 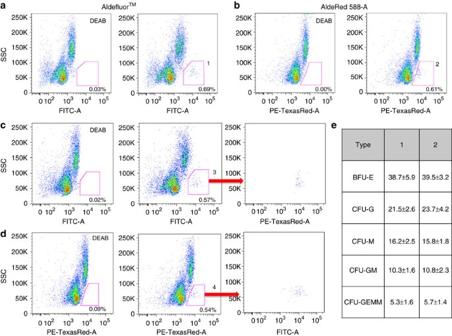Figure 3: AldeRed 588-A successfully enables isolation of ALDHhiHSCs from human cord blood mononuclear cells. (a) ALDEFLUOR, (b)AldeRed 588-A, (c,d) double staining with ALDEFLUOR andAldeRed 588-A. Red boxes represent gating for sorting ALDHhicells (1and2). Numbers at the bottom represent percentage of gated cells. ALDHhicells (3and4) were present in the other channels. Figure 3: AldeRed 588-A successfully enables isolation of ALDH hi HSCs from human cord blood mononuclear cells. ( a ) ALDEFLUOR, ( b ) AldeRed 588-A , ( c , d ) double staining with ALDEFLUOR and AldeRed 588-A . Red boxes represent gating for sorting ALDH hi cells ( 1 and 2 ). Numbers at the bottom represent percentage of gated cells. ALDH hi cells ( 3 and 4 ) were present in the other channels. Full size image Table 1 Colony-forming cell assays with isolated ALDH hi cells ( 1 and 2 ). Full size table Fractionation of ALDH pos cells from mice expressing eGFP Since the BODIPY fluorophore for the ALDEFLUOR reagent emits green light, cells harvested from transgenic mice expressing green-fluorescent tags cannot be studied with this standard reagent. To test whether one could use AldeRed 588-A with cells from a transgenic mouse expressing an enhanced green-fluorescent protein (eGFP) tag, we attempted to enrich ALDH int murine haematopoietic stem and progenitor cells (HSPCs) among eGFP-expressing bone marrow (BM) cells isolated from transgenic notch reporter ( TNR (transgenic notch reporter) , Tg(Cp-EGFP)25Gaia ) mice [10] . The TNR mice express eGFP in cells with active notch signalling attributed to the C promoter (Cp)-binding factor 1-binding site upstream of the eGFP gene. We chose to study the TNR mice for two reasons, both related to biologically relevant systems to assess the utility of our reagent. First, although it is known that murine HSPCs demonstrate high notch signalling activity [10] , the function of notch signalling in maintenance of HSPCs is controversial [12] , [13] . Second, there has been disagreement with respect to using ALDH as a marker for murine HSPCs. While the ALDEFLUOR reagent has been used to isolate functional murine HSPCs [14] , [15] , one group reported that Aldh1a1 -deficient mice had normal haematopoiesis and functional HSPCs [16] . The TNR mice provide a suitable model to test red-fluorescent AldeRed 588-A for its ability to fractionate cells according to ALDH activity from eGFP pos notch active cells. We isolated BM cells from 5- to 6-week-old TNR mice and stained them with AldeRed 588-A . We fractionated those cells into five different populations: eGFP neg /ALDH hi 1 , eGFP pos /ALDH hi 2 , eGFP neg /ALDH int 3 , eGFP pos /ALDH int 4 and eGFP neg /ALDH lo 5 ( Fig. 4b ). To examine in which population HSPCs reside, we isolated each population and performed colony forming cell assays. We found that the eGFP pos /ALDH int cell population 4 formed colonies CFU-GEMM, CFU-GM, CFU-M and BFU-E, while none of the other cell populations formed a single colony ( Fig. 4e ). To verify that HSPCs reside within the eGFP pos /ALDH int population, we performed multicolour FACS analysis for lineage − /c-Kit + /Sca1 + (LKS) HSPCs in addition to ALDH staining using AldeRed 588-A . LKS cells were present within the eGFP pos /ALDH int population 4 ( Fig. 4c ). In addition, the red fluorescence of the LKS cells shifted when compared with DEAB-treated control, indicating that LKS cells possess active ALDH ( Fig. 4d ). 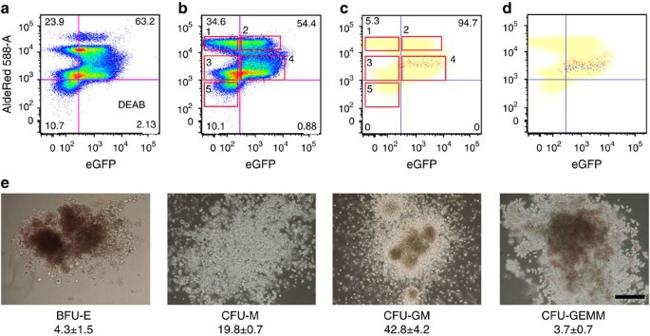Figure 4: AldeRed 588-A can enable the fractionation of ALDHposcells from BM cells from mice that express eGFP. (a–d) Fractionation of BM cells based on eGFP expression andAldeRed 588-Auptake levels (numbers represent percentage of each quadrant fraction). (a) DEAB control. (b) Sorting of BM cells into five populations (red box) for colony forming assays of sorted cells. (c,d) Enrichment of LKS HSPCs within BM cells. LKS cell populations (red dots for untreated (c) and blue dots for DEAB-treated cells (d)) were back-gated on total BM cells (yellow). The gating strategy (red boxes) for the colony-forming assay inbis superimposed on LKS and BM cell populations (c). (e) Representative photos of colony-forming cell assays. BFU-E: burst forming unit-erythroid; CFU-GEMM: colony forming unit-granulocyte, erythrocyte, monocyte, megakaryocyte; CFU-GM: colony forming unit-granulocyte, monocyte; CFU-M: colony forming unit-megakaryocyte. Numbers represent colonies formed per 20,000 eGFPpos/ALDHintcells (4)± s.d.,n=6. Size bar: 100 μm. Figure 4: AldeRed 588-A can enable the fractionation of ALDH pos cells from BM cells from mice that express eGFP. ( a – d ) Fractionation of BM cells based on eGFP expression and AldeRed 588-A uptake levels (numbers represent percentage of each quadrant fraction). ( a ) DEAB control. ( b ) Sorting of BM cells into five populations (red box) for colony forming assays of sorted cells. ( c , d ) Enrichment of LKS HSPCs within BM cells. LKS cell populations (red dots for untreated ( c ) and blue dots for DEAB-treated cells ( d )) were back-gated on total BM cells (yellow). The gating strategy (red boxes) for the colony-forming assay in b is superimposed on LKS and BM cell populations ( c ). ( e ) Representative photos of colony-forming cell assays. BFU-E: burst forming unit-erythroid; CFU-GEMM: colony forming unit-granulocyte, erythrocyte, monocyte, megakaryocyte; CFU-GM: colony forming unit-granulocyte, monocyte; CFU-M: colony forming unit-megakaryocyte. Numbers represent colonies formed per 20,000 eGFP pos /ALDH int cells ( 4 )± s.d., n =6. Size bar: 100 μm. Full size image Staining of ALDH pos murine pancreatic stem cells As an additional example of the utility of AldeRed 588-A , we tested its capacity for identifying ALDH pos cells in vitro with fluorescence microscopy. We have previously shown that a subset of murine pancreatic centroacinar and terminal duct (CA/TD) cells expressing abundant Aldh1a1 and Aldh1a7 can be imaged and isolated using the ALDEFLUOR reagent [17] . We have also shown that the isolated CA/TD cells exhibited characteristics of murine pancreatic progenitor cells. Using AldeRed 588-A and the ALDEFLUOR reagent, we stained isolated murine CA/TD cells and examined them under fluorescence microscopy. Both red and green substrates successfully stained CA/TD cells without overlap between the detection filters for each reagent ( Fig. 5a,b ). Upon co-staining, red and green signals overlapped, indicating ALDH specificity ( Fig. 5c and Supplementary Fig. 8 ). 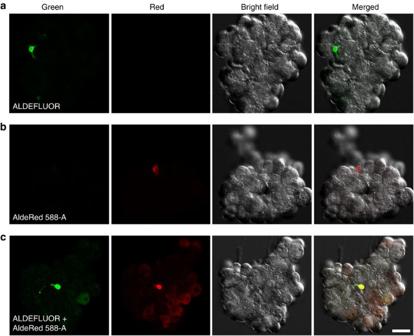Figure 5: AldeRed 588-A stains ALDHhimurine pancreatic centroacinar and terminal duct (CA/TD) cells. Confocal microscopic images of murine pancreatic CA/TD cells stained with the ALDEFLUOR reagent (a),AldeRed 588-A(b) and co-stained with both reagents (c). Size bar: 20 μm. Figure 5: AldeRed 588-A stains ALDH hi murine pancreatic centroacinar and terminal duct (CA/TD) cells. Confocal microscopic images of murine pancreatic CA/TD cells stained with the ALDEFLUOR reagent ( a ), AldeRed 588-A ( b ) and co-stained with both reagents ( c ). Size bar: 20 μm. Full size image Stem cells are important new reagents in biomedical research. They can provide experimental models for target discovery [18] or toxicity testing [19] and can be used as tools for screening drugs and in developing therapies for a host of disorders [20] , [21] . Stem cells can provide a direct source of materials for regenerative medicine [22] . The ability to prepare pure, undamaged and functionally active stem cells is the critical first step for all such applications. Isolation of stem cells is generally carried out by selection with monoclonal antibodies that recognize stem cell-specific cell surface markers or by utilizing functional markers of stem cell activity, such as elevated expression of multidrug efflux pumps [23] and ALDH [8] . Combinations of multiple markers, often requiring multiple steps of selection, are used to isolate rare stem cells from heterogeneous cell populations. A brief, single-step isolation method would be preferred to minimize loss of and damage to rare stem cells. We present a red-shifted agent that provides additional flexibility for utilizing ALDH as a marker for stem cell isolation. The ALDEFLUOR assay, the only commercially available method to detect and isolate functionally active ALDH pos cells, depends on differences in fluorescence intensity obtained for the cellular retention of green-fluorescent substrate in the presence and absence of the ALDH inhibitor, DEAB. As a red-shifted substrate for ALDH, AldeRed 588-A will enable isolation of stem cells from a green-fluorescent background, which is increasingly prevalent as many genes—including those in transgenic models—are tagged with eGFP. In addition, since many cells demonstrate autofluorescence in the green region of the spectrum [24] , there is a chance of false-positive results from stem cell isolation with ALDEFLUOR. AldeRed 588-A could provide an additional way to confirm the purity of ALDH-active cells when used in conjunction with ALDEFLUOR. In order to act as a functional probe for ALDH, a compound should possess three characteristics: an aldehyde moiety that can serve as a substrate for ALDH; suitable hydrophobicity for free diffusion into cells; and capacity for subsequent trapping within the cytoplasm after conversion of the aldehyde into the corresponding acid by ALDH. Our initial choice for three red fluorophores was based on their lack of charged groups, such as sulphonic acid or carboxylic acid, found in other commercial dyes such as the Cy series, Alexa Fluor or IRDye. Those charged groups may prevent the substrate from penetrating the plasma membrane, limiting access to cytoplasmic ALDH. Of the three compounds tested, only AldeRed 588-A met all the three criteria. The degree of trapping is particularly challenging to control. Vaidyanathan et al. [25] reported two radiolabelled ALDH substrates that could be converted into the acid form by the purified enzyme. Both substrates, however, failed to accumulate inside of cells with high ALDH activity when compared with the DEAB control. The authors discussed the lack of appropriate physical characteristics (hydrophobicity) as a possible cause. AldeRed 588-A has a red-shifted emission spectrum and possesses physical properties that enable it to function as a probe for ALDH in vivo . Although AldeRed 588-A would provide a tool to researchers using green-fluorescent materials, it has a limitation for multicolour application—for example, 14 colour sorting with flow cytometry—due to its broad emission spectrum ( Supplementary Figs 2–4 ). AldeRed 588-A would, however, allow for six colour sorting with the LSR II (BD Biosciences) FACS equipped with four lasers and 14 emission filters. Nevertheless, we continue to search for a fluorescent substrate for ALDH with a narrow emission spectrum to enable enhanced multicolour sorting. We initially chose cell lines known to express abundant, functional ALDH homogeneously for cell-based validation of our candidate substrates ( Fig. 2 ). We then tested whether AldeRed 588-A could isolate ALDH hi cells among a mixture of heterogeneous cell populations using mononuclear cells from human cord blood. Human HSCs are known to express high levels of ALDH, and the ALDEFLUOR reagent has been used to purify ALDH hi HSCs via simple staining and sorting [8] , [26] . AldeRed 588-A demonstrated essentially the same efficiency as ALDEFLUOR for isolating ALDH hi HSCs and can be used simultaneously ( Figs 3c,d and 5c , Supplementary Figs 6 and 8 ). Such co-staining could be used to increase further the specificity of the detection of true ALDH pos cells, particularly in the context of a green-fluorescent background. It has been reported that Aldh1a1 is unnecessary for murine HSPC function but also that Aldh1a1 −/− BM cells stain positive with the ALDEFLUOR reagent, confusing the issue of ALDH function in HSPCs [16] . Recently, Garaycoechea et al. [27] demonstrated that murine HSPCs could be stained using ALDEFLUOR by virtue of the activity of ALDH2, which plays a role in detoxifying acetaldehyde. Our results suggest that murine HSPCs possess ALDH activity. It will be interesting to examine whether AldeRed 588-A exhibits a similar staining pattern to ALDEFLUOR with respect to HSPCs of Aldh1a1 −/− and Aldh2 −/− mice. We anticipate that AldeRed 588-A will provide increased flexibility to study a variety of different aspects of ALDH, particularly in the presence of a green-fluorescent background. Cell Lines and animals The K562 human chronic myelogenous leukemia cell line was purchased from American Type Culture Collection (CLL-243) and maintained in suspension in IMDM media supplemented with 10% fetal bovine serum (FBS). The murine leukemia cell lines L1210 (ALDH low ) and L1210/cpa (ALDH hi ) were provided by Dr Richard J. Jones (Johns Hopkins University) and maintained in suspension in RPMI 1640 supplemented with 10% FBS. All cells were grown at 37 °C in a humidified incubator with 5% CO 2 . All animal experiments were performed in accordance with protocols approved by the Johns Hopkins University Animal Care and Use Committee. Reagents and analyses BODIPY 576/589 succinimidyl ester and BODIPY 650/665 succinimidyl ester were purchased from Life Technologies Inc. (Grand Island, NY). ( E )-4-(4-(dimethylamino)styryl)-1-(3-isothiocyanatopropyl)pyridin-1-ium chloride 1 was synthesized analogously to the previously reported di-butyl analogue [28] . Chemicals and solvents for synthesis and high-performance liquid chromatography (HPLC) were acquired from Sigma-Aldrich (Milwaukee, WI, USA) or Fisher Scientific (Pittsburgh, PA, USA), and used without further purification. HPLC was performed on an Agilent Prostar System equipped with a 325 Variable wavelength detector and controlled by Galaxie Software using a Phenomenex 4.6 × 250 mm Luna C18, 10-μ column. AldeRed 493 aldehyde diethyl acetal ( Supplementary Fig. 9a,b ) and AldeRed 493-A ( Supplementary Fig. 9c,d ) were chromatographed using Method 1. AldeRed 588 aldehyde diethyl acetal ( Supplementary Fig. 10a,b ), AldeRed 588-A ( Supplementary Fig. 10c,d ), AldeRed 659 aldehyde diethyl acetal ( Supplementary Fig. 11a,b ), AldeRed 659-A ( Supplementary Fig. 11c,d ), BODIPY-aminoacetaldehyde-diethyl acetate ( Supplementary Fig. 12a,b ), and activated ALDEFLUOR Reagent ( Supplementary Fig. 12c,d ) were chromatographed using Method 2. Method 1: Solvent A: 100% water; Solvent B: 100% methanol; 0–5 min 100% A, 5–25 min linear gradient from 100% A to 100% B, 25–30 min 100% B, 30–35 min linear gradient from 100% B to 100% A, 35–38 min 100% A, 2 ml min −1 . Method 2: Solvent A: 100% water; Solvent B: 100% acetonitrile; 0–20 min linear gradient from 90% A/10% B to 10% A/90% B; 20–25 min 10% A/90% B, 25–30 min linear gradient from 10% A/90% B to 90% A/10% B, 2 ml min −1 . 1 H NMR spectra were obtained on a Bruker Avance 400 MHz Spectrometer. High-resolution mass spectra were obtained by the University of Notre Dame Mass Spectrometry & Proteomics Facility (Notre Dame, IN, USA) using ESI either by direct infusion on a Bruker micrOTOF-II or by LC elution via an ultra-high pressure Dionex RSLC with C18 column coupled with a Bruker micrOTOF-Q II. The excitation and emission profiles of synthesized products were measured using a spectrofluorophotometer (Shimadzu, RF-5301pc, Columbia, MD, USA). Synthesis of AldeRed 493 amino acetal aldehyde diethyl acetal 4 Aminoacetaldehyde diethyl acetal (0.024 mmol, 3 μl) was added to a solution of ( E )-4-(4-(dimethylamino)styryl)-1-(3-isothiocyanatopropyl)pyridin-1-ium chloride 1 (3.6 mg, 0.01 mmol in 1 ml of dimethylformamide) and 5 μl of triethylamine and was mixed by stirring for 30 min in the dark. Five microlitres of water were added and the resulting solution was extracted with ether (2 × 5 ml). Water in the aqueous phase was evaporated under vacuum and the residue was purified by passing through a small C18 column, eluted with 1:1 water/acetonitrile. Yield: 1.8 mg, 0.004 mmol, 40%. 1 H NMR(400 MHz, dimethylsulphoxide-d 6 ): δ =1.10 ( t , 6H, J =7.6 Hz); 2.09–2.13 (m, 2H); 3.0 (s, 6H); 3.4–3.5 (m, 6H); 3.55–3.62 (m, 2H); 4.43 ( t , 2H, J =6.8Hz); 4.5–4.6(m, 1H); 6.77 (d, 2H, J =8.8Hz); 7.15(d, 1H, J=16.4Hz); 7.58(d, 2H, J=8.4 Hz); 7.90(d, 1H, J=15.6 Hz); 8.04(d, 2H, J=6.8 Hz); 8.74 (d, 2H, 6.8 Hz). HRESI-MS C 25 H 37 N 4 O 2 S + calcd 457.2632; found 457.2632 ( Supplementary Fig. 13 ). Synthesis of AldeRed 588 aldehyde diethyl acetal 5 Aminoacetaldehyde diethyl acetal (0.024 mmol, 3 μl) was added to BODIPY 576/589 succinimidyl ester 2 (5 mg, 0.012 mmol in 1 ml of tetrahydrofolate (THF)) and mixed by stirring for 30 min in the dark. After evaporating THF, AldeRed 588 aldehyde diethyl acetal 5 was purified with flash column chromatography using ethyl acetate/hexane (1:1) as an eluent to give 3.8 mg, 0.0086, mmol 75% yield. 1 H NMR (400 MHz, CDCl 3 ): δ =1.16 ( t , 6H, J =7 Hz); 2.65 ( t , 2H, J =7.2 Hz); 3.31 ( t , 2H, J =7.2 Hz); 3.37 (t, 2H, J =5.6 Hz); 3.48 (m, 2H); 3.65 (m,2H); 4.43 (t, 1H, 5.6 Hz); 5.82 (br, 1H); 6.27 (d, 1H, 3.6=3.6 Hz); 6.36 (br, 1H); 6.81 (d, 1H, J =4 Hz); 6.85 (d, 1H, 4.4 Hz); 6.96 (s, 1H); 6.97 (s, 1H), 7.02 (d, 1H, J =4.4 Hz); 7.16 (s, 1H). HRESI-MS C 22 H 28 BF 2 N 4 O 3 calcd 445.4222; found 445.4222 ( Supplementary Fig. 13 ). Synthesis of AldeRed 659 aldehyde diethyl acetal 6 Aminoacetaldehyde diethyl acetal (0.016 mmol, 2 μl) was added to BODIPY 650/665 succinimidyl ester 3 (5 mg, 0.0078, mmol in 1 ml of THF) and was mixed by stirring for 30 min in the dark. After evaporating THF, AldeRed 659 aldehyde diethyl acetal 6 was purified with flash column chromatography using ethyl acetate/hexane (1:1) as an eluent to give 3.5 mg, 0.0053, mmol, 70% yield. 1 H NMR (400 MHz, CDCl 3 ): δ =1.19 ( t , 6H, J =7.8 Hz); 1.33–1.37 (m, 2H), 1.5–1.58 (m, 2H); 1.6–1.68 (m, 2H); 2.16 ( t , 2H, J =7.8 Hz); 3.31–3.38 (m, 4H); 3.46–3.55 (m, 2H); 3.62–3.71 (m, 2H); 4.46 ( t , 1H, J =5.2 Hz); 4.51 (s, 2H); 5.65 (br, 1H); 6.36–6.39 (m, 1H); 6.57–6.62 (m, 1H); 6.83–6.88 (m, 2H); 6.89 (d, 1H, J =4 Hz); 6.92–6.98 (m, 4H); 7.0 (d, 1H, J =4 Hz); 7.18 (m, 1H); 7.50–7.58 (m, 3H). HRESI-MS C 35 H 43 BF 2 N 5 O 5 calcd 662.3326; found: 662.3326 ( Supplementary Fig. 13 ). Preparation of aldehyde derivatives All diethyl acetal precursors to the final aldehyde derivatives were dissolved in 100% dimethylsulphoxide at 5 mM and stored at −20 °C in stock solutions. Immediately before the assay, a 25-μl aliquot of each stock solution was deprotected by adding the same volume of 2 N HCl followed by incubation for 30 min at room temperature. The resulting reaction mixtures were neutralized by adding 350 μl of assay buffer (phosphate-buffered saline supplemented with 1% FBS and 50 μM verapamil). Isolation of AldeRed 588-A In order to characterize AldeRed 588-A produced upon hydrolysis, AldeRed 588 aldehyde diethyl acetal 5 (0.5 mg in 300 μl) was mixed with 300 μl of 2 N HCl and incubated for 30 min at room temperature. The reaction mixture was then diluted with 2 ml of water. The clear purple solution was injected into the HPLC. The purification of AldeRed-588-A was performed using an Agilent 1260 infinity preparative HPLC system equipped with a Phenomenex Luna C18, 10-μ column and a flow rate of 10 ml min −1 . The desired product eluted at 3.3 min with acetonitrile/water (40/60) and collected. (The solvent front eluted at 1.1 min.) The collected fraction was frozen at −78 ° C immediately and lyophilized to dryness. Approximately 0.4 mg of AldeRed-588-A was obtained as a dark powder. HRESI-MS C 18 H 18 BF 2 N 4 O 2 calcd 371.1485; found: 371.1489 ( Supplementary Fig. 14 ). In vitro fluorescence uptake assay for ALDH activity One million cells were resuspended in assay buffer and 5 μl of the corresponding aldehyde (ALDEFLUOR, AldeRed 493-A , AldeRed 588-A or AldeRed 659-A ) was added to the suspension. In each case a 0.5-ml aliquot of the suspension was immediately added to a 5-ml polystyrene round bottom tube (BD Biosciences) containing 5 μl of DEAB (STEMCELL Technologies Inc., Vancouver, BC, Canada). Cells were incubated in a water bath at 37 °C for 30 min followed by washing with 4 ml of cold assay buffer once. Cells were resuspended in cold assay buffer (5 × 10 5 per 200 μl) and stored on ice until analysed. Stained cells were analysed with FACS LSR II (BD Biosciences) equipped with four lasers (405, 488, 532 and 633 nm) and 14 emission filters. All three candidate ALDH substrates were tested on all 15 filters. AldeRed 588-A was also tested on a FACSCalibur (BD Biosciences) with 488-nm blue laser and phycoerythrin (PE) filter. Isolation of ALDH hi human HSCs Frozen human cord blood mononuclear cells were purchased from ALLCELLS (Alamenda, CA, USA). Cells were thawed according to the provider’s instructions immediately before use followed by re-suspension in assay buffer (1 × 10 6 cells ml −1 ). The staining procedure for ALDEFLUOR and AldeRed 588-A was same as described above for the in vitro fluorescence uptake assay. ALDH hi cells were sorted into RPMI supplemented with 10% FBS using FACSAria (BD Biosciences) equipped with four lasers (405, 488, 532 and 633 nm) and 14 emission filters. Five hundred ALDH hi cells were plated in 1 ml of Methocult H4435 (STEMCELL Technologies Inc.) and incubated in a humidified incubator at 37 °C with an atmosphere of 5% CO 2 for 1 week. Colonies formed were counted 1 week later and photographed using a Nikon TE-200 inverted microscope. Enrichment of HSCs from BM cells of TNR mice TNR mice [ Tg(Cp-EGFP)25Gaia ] were provided by Dr Shyam Biswal (Johns Hopkins School of Public Health). BM cells from 6-week-old male mice were harvested by repeatedly flushing the femur, tibia and pelvis with a 26Gx5/8 needle. Red blood cells were depleted using RBC lysis buffer (BioLegend, San Diego, CA, USA) according to the manufacturer’s instructions. Cells were stained with AldeRed 588-A and sorted into five populations (eGFP neg /ALDH pos , eGFP neg /ALDH int , eGFP neg /ALDH hi , eGFP pos /ALDH int, and eGFP pos /ALDH hi ) using FACS Aria (BD Biosciences) with fluorescein isothiocyanate and PE-Texas Red filters for eGFP and AldeRed 588-A , respectively. Twenty thousand cells from each population were plated in 1 ml of Methocult M3434 (STEMCELL Technologies Inc.) and incubated in a humidified incubator at 37 °C and in an atmosphere of 5% CO 2 for 1 week. Colonies formed were counted 1 week later and photographed using a Nikon TE-200 inverted microscope. A mouse haematopoietic lineage cocktail (eFluor450, eBiosciences) containing anti-mouse Ly-6A/E (PE-Cy7, BioLegend) and anti-mouse CD117 (APC-Cy7, BioLegend) was used according to the manufacturer’s instruction to stain and isolate LKS cells using LSR II. Microscopic ALDH staining of murine pancreatic cells Mouse pancreatic acinar preparation was performed as previously described [29] . Briefly, adult CD1 mouse pancreas was harvested and digested in 1 mg ml −1 collagenase-P (Roche, Indianapolis, IN, USA) at 37 °C in a water bath for 15 min. The collagenase-P reaction was terminated by the addition of ice-cold HBSS with 5% FBS. Following multiple washes, collagenase-digested pancreatic tissue was filtered through a 500-μm polypropylene mesh (Spectrum Laboratories, Rancho Dominguez, CA, USA). The resulting acinar units were resuspended in 20 ml of ALDEFLUOR assay buffer (STEMCELL Technologies Inc.). To label the cells with fluorescent agent, 5 μl of green ALDEFLUOR substrate and 5 μl of AldeRed 588-A were used per 1 ml of ALDEFLUOR assay buffer. Cell staining proceeded at 37 °C for 50 min. A DEAB control reaction was performed in parallel. Samples were placed in ice to terminate the reaction. Live cell imaging was performed on a Nikon A1 Confocal system (Nikon Instruments Inc., Melville, NY, USA). The optical configuration was optimized for the DEAB control sample eliminating possible signal in green and red channels. All images were taken using the same optical setting. How to cite this article: Minn, I. et al. A red-shifted fluorescent substrate for aldehyde dehydrogenase. Nat. Commun. 5:3662 doi: 10.1038/ncomms4662 (2014).